Multicomponent double Mannich alkylamination involving C(sp2)–H and benzylic C(sp3)–H bonds Alkylamines are ubiquitous in pharmaceuticals, materials and agrochemicals. The Mannich reaction is a well-known three-component reaction for preparing alkylamines and has been widely used in academic research and industry. However, the nucleophilic components in this process rely on C(sp 2 )−H and activated C(sp 3 )−H bonds while the unactivated C(sp 3 )−H bonds involved Mannich alkylamination is a long-standing challenge. Here, we report an unprecedented multicomponent double Mannich alkylamination for both C(sp 2 )−H and unactivated benzylic C(sp 3 )−H bonds. In this process, various 3-alkylbenzofurans, formaldehyde and alkylamine hydrochlorides assemble efficiently to furnish benzofuran-fused piperidines. Mechanistic studies and density functional theory (DFT) calculations revealed a distinctive pathway that a multiple Mannich reaction and retro-Mannich reaction of benzofuran and dehydrogenation of benzylic C(sp 3 )−H bonds were key steps to constitute the alkylamination. This protocol furnishes a Mannich alkylamine synthesis from unusual C–H inputs to access benzofuran-fused piperidines with exceptional structural diversity, molecular complexity and drug-likeness. Therefore, this work opens a distinctive vision for the alkylamination of unactivated C(sp 3 )−H bonds, and provides a powerful tool in diversity-oriented synthesis (DOS) and drug discovery. Alkylamines are fundamental compounds in pharmaceuticals, materials, and agrochemicals [1] , [2] . For their synthesis, the Mannich reaction represents one of the most efficient approaches to access these molecules [3] . Discovered in 1912, the Mannich reaction is a prototypical three-component reaction that rapidly assembles a resonance-stabilized carbon nucleophile, an aldehyde (or ketone) and an amine to afford alkylamines. The mechanistic manifold involves iminium ion formation for sequential attack by a nucleophile. Owing to the readily accessible feedstocks, simple manipulation, and privileged product formation, the Mannich reaction is well suited for diversity-oriented synthesis (DOS) applicable in drug discovery, and its utility is demonstrated in alkaloid synthesis and the development of the antiulcer drug Ranitidine [4] , [5] , [6] , [7] , [8] , [9] , [10] , [11] . Recently, the asymmetric version of Mannich reaction has attracted much interests [12] , [13] , [14] , [15] , [16] , [17] , [18] , [19] , [20] , [21] , [22] . Despite these advances, the nucleophilic components of the Mannich reaction rely on Brønsted-acidic carbonyl C(sp 3 )−H bonds (Fig. 1a ) and C(sp 2 )−H centers of electron-rich arenes (Fig. 1b ) [23] , [24] , while the development of a Mannich reaction using unactivated C(sp 3 )–H bonds has remained a formidable challenge. Fig. 1: Overview of Mannich reaction. a Classical Mannich reaction involving activated C(sp 3 )−H bond. b Mannich reaction involving C(sp 2 )−H bond of electron-rich arenes. c This work of double Mannich alkylamination for both C(sp 2 )−H and unactivated benzylic C(sp 3 )−H bond. Full size image As noted, the wide prevalence of alkylamines in small molecule biological probes, pre-clinical candidates, and approved drugs is owing to their favorable physical and pharmacological properties [25] , [26] . In particular, cyclic alkylamines can enhance structural rigidity, thus improving target selectivity and druggability. For example, the cyclic six-membered piperidines represent the most commonly used nitrogen heterocycles among U.S. FDA-approved pharmaceuticals (Fig. 2 ). As a highly relevant synthetic strategy, the double Mannich reaction based on enolizable C−H bonds provides straightforward access to cyclic alkylamines. This was exemplified by Robinson for the facile synthesis of tropinone [27] . To engage unactivated C(sp 3 )−H bonds in this process would significantly expand the synthetic toolbox for the assembly of cyclic alkylamines and drug candidates. Based on serendipitous findings, herein, we report on the discovery of a multicomponent double Mannich reaction for both C(sp 2 )−H and unactivated benzylic C(sp 3 )−H bonds (Fig. 1c ). In this process, various 3-alkylbenzofurans, formaldehyde, and primary alkylamine hydrochlorides assemble efficiently to furnish diverse benzofuran-fused piperidines. In addition, many bioactive molecules could be applicable in this protocol to prepare their analogs. Fig. 2: Pharmaceutical relevant examples of piperidines. Piperidine is widely existed in natural products and serves as the most commonly used nitrogen heterocycle among U.S. FDA-approved pharmaceuticals. Full size image Reaction design and optimization for double Mannich reaction As mentioned above, the challenge for unactivated C(sp 3 )−H bonds to involve in Mannich reactions is attributed to their difficult deprotonation and therefore non-nucleophilic properties. In continuation of our interest in multi-component reactions and drug discovery [28] , [29] , [30] , [31] , we hypothesized that the benzylic C(sp 3 )−H bond might possess sufficient reactivity through the electronic effect of (hetero)arenes, thus enabling Mannich type alkylamination. After considerable exploration and optimization of conditions, we realized this hypothesis using electron-rich benzofurans as heteroaryl substrates. 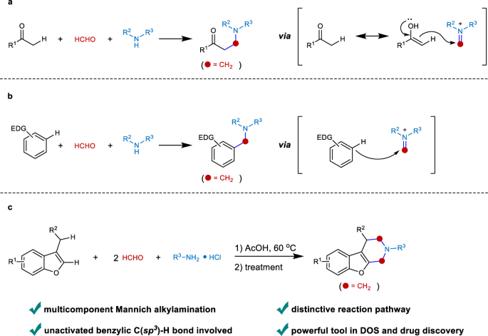Fig. 1: Overview of Mannich reaction. aClassical Mannich reaction involving activated C(sp3)−H bond.bMannich reaction involving C(sp2)−H bond of electron-rich arenes.cThis work of double Mannich alkylamination for both C(sp2)−H and unactivated benzylic C(sp3)−H bond. As shown in Table 1 , the model reaction was explored with benzofuran 1a , formaldehyde 2 , and glycine methyl ester hydrochloride 3a . In the solvent of acetic acid (AcOH), these three components were mixed in a one-pot and kept at 60 °C for 3 h (entries 1–6). The amounts of 2 and 3a were varied while a major product was formed and identified as benzofuran-fused piperidine 4a in 74% yield (entry 6). This indicated an efficient double Mannich alkylamination involving both the benzylic C(sp 3 )−H bond and the aryl C(sp 2 )−H bond, furnishing the cyclic amine. Increasing the reaction temperature would decrease the yield (entries 7–8) and only 25% yield could be obtained when conducted at room temperature (entry 9). The survey of solvents showed that acetonitrile (CH 3 CN) worked equally well (entry 10), while the utilization of isopropanol, hexafluoroisopropanol (HFIP), and HFIP/AcOH would give inferior results (entries 11–13). Variation of 3a to glycine methyl ester would lead to a decreased yield (entry 14). Conducting this reaction on 5 mmol scales could afford 4a with slightly improved yield (entry 15), thus underscoring the scalability of this process. Table 1 Reaction optimization a . Full size table Substrate scope in the synthesis of benzofuran-fused piperidines Under the optimized conditions, we examined the substrate scope of this three-component double Mannich alkylamination. Various amino acid derivatives, including glycine, l -alanine, l -phenylalanine, l -valine, l -leucine, l -serine, l -cysteine, l -methionine, l -aspartic acid, l -glutamic acid, l -tyrosine, and l -isoleucine, all reacted smoothly with benzofuran 1a and formaldehyde 2 to furnish the corresponding fused piperidines in moderate to good yields ( 4a - 4o ) (Fig. 3 ). The structure of 4b and 4n was confirmed by X-ray analysis. Notably, the chirality and functionalities of the amino acids were retained in this process thus bestowing versatile physical and pharmacological properties on the products (see Supplementary Information ). Besides, numerous primary amines hydrochlorides could engage in this process at 90 °C, and benzyl, alkene, alkyne, trifluoromethyl, ester, alcohol, sulfone, amino and bromoalkyl functionalities were well tolerated. This offers ample opportunity for further functionalization towards drug discovery and small molecule biological probe development. The structure of 4r was confirmed by X-ray analysis. Moreover, three-, four-, five-, and six-membered ring-substituted amines were used to furnish the products in moderate to good yields ( 4z - 4ac ). Furthermore, a primary amine substituted with a quaternary carbon center was used, and also in this case the cyclization took place, giving 4ad in moderate yield. Additionally, the late-stage modification of drug derivatives could be achieved using this method. For instance, the important neurotransmitter GABA (γ-aminobutyric acid) methyl ester hydrochloride 3ae , the antiepileptic drug Pregabalin methyl ester hydrochloride 3af , the monoamine oxidase inhibitor Tranylcypromine hydrochloride 3ag , and the antiarrhythmic drug Mexiletine hydrochloride 3ah , could all be efficiently modified under this protocol to produce the corresponding piperidine-hybrids in moderate yields ( 4ae - 4ah ). In addition, the utilization of CH 3 CN as solvent also works well with extended reaction time. Fig. 3: Substrate scope of amines. Condition A (for 3a – 3o ): 1a (0.2 mmol), 2 (0.8 mmol), 3 (0.4 mmol) in AcOH (2 mL) at 60 °C, 3 h; Condition B (for 3p - 3ah ): 1a (0.2 mmol), 2 (1.6 mmol), 3 (0.8 mmol) in AcOH (2 mL) at 90 °C, 30 mins. Yields refer to isolated products. N(Phth) = N -phthalimide. a CH 3 CN (2 mL) as solvent, 8 h. Full size image With respect to heteroarenes, a variety of electron-rich 3-alkylbenzofurans underwent the three-component double Mannich alkylaminaion efficiently, occurring at the 2-position of the benzofuran and the benzylic moiety (Fig. 4 ). Diverse functionalized substituents were tolerated in this process, including alkyloxy, allyloxy, propargyloxy, hydroxy, alkylthio, alkyl, chloro, bromo, and boronate ( 5a - 5m ). It should be noted that these functionalities not only bestow the products with remarkable structural diversity and favorable physical properties, but also provides ample potential for further derivatization. For example, the boronate compound 5m might be transformed to a variety of molecules through Suzuki coupling reaction and Chan-Lam coupling reaction. When benzofurans with a substituted benzyl group like 3-ethyl, 3-(2-phenyl)ethyl, 3-(4-hydroxy)butyl, and 3-(4-amino)butyl were used, interestingly, the double Mannich reaction proceeded well to give the poly-substituted and functionalized piperidines in excellent yields ( 5n - 5r ). Besides, the hydroxy and amino group in the substituted chain would offer numerous late-stage functionalization opportunities. Moreover, compound 5r was further subjected to a Huisgen click reaction to yield a triazole derivative 5s , whose structure was confirmed by X-ray analysis. Considering that the piperidines are prevalent motifs in natural products as well as pharmaceuticals and are important synthetic targets for drug discovery and development [32] , this process provides an efficient and direct approach to establish libraries with high drug-likeness, broad chemical space, and modifiable physicochemical properties. Fig. 4: Substrate scope of heteroarenes. Reactions were carried out under condition A. Yields refer to isolated products. N(Phth) = N -phthalimide. a 3a was replaced with propargylamine hydrochloride under condition B. b 5s was prepared from 5r via click reaction. Full size image Mechanistic investigation Next, mechanistic studies were conducted to gain insights into the mechanism. (i) Control reactions (Fig. 5a ): when this three-component reaction was carried out at room temperature, the common Mannich reaction occurred to deliver a mixture of 6 and 7 ( 6 , 28% isolated yield; 7 , 70% isolated yield). 6 was a Mannich alkylamination product at the 2-position of benzofuran, and 7 was a dialkylated Mannich amine. Interestingly, 6 and 7 could interconvert under this condition (see Supplementary Information ). Furthermore, they could react with 2a and 3 to deliver product 4a in yields of 93% and 68%, respectively, indicating that 6 and 7 were probable intermediates of this process. (ii) Kinetic isotopic effect experiments (Fig. 5b ): benzylic deuterium-labeled [D 3 ]-1a was prepared and combined with 2a and 3 under standard reaction conditions, leading to the corresponding product [D 2 ]-4a in 54% yield. Additionally, a kinetic isotope effect (KIE) study was carried out and a primary KIE value of 1.8 was observed, suggesting that the C(sp 3 )−H bond cleavage might be involved in the rate-limiting step. (iii) Radical-probe experiments (Fig. 5c ): a radical scavenger was added to the one-pot reaction including 6 , 2 , and 3a to probe the involvement of a radical intermediate. Ether the addition of TEMPO (2,2,6,6-tetramethylpiperidinooxy, 1 equiv.) or BHT (butylated hydroxytoluene, 1 equiv.) did not suppress the Mannich reaction. In addition, the cyclopropane-containing substrate 1 s was prepared and subjected to the reaction, and a piperidine product 5t was isolated in 87% yield with cyclopropane retaining. These suggested exclusion of radical intermediates in this reaction [33] , [34] , [35] , [36] , [37] , [38] , [39] , [40] , [41] , [42] , [43] , [44] . Fig. 5: Mechanistic studies. a Control reaction. b Kinetic isotope effect experiments. c Radical-probe experiments. Full size image On the basis of these observations, a plausible mechanism was proposed with starting materials 1a , formaldehyde 2 , and methyl glycinate hydrochloride 3a as model substrates (Fig. 6a ). Initially, the electron-rich 3-methylbenzofuran 1a , formaldehyde 2 , and methyl glycinate hydrochloride 3a undergo the first Mannich alkylamination to deliver intermediate A (compd. 6 ). A undergoes the secondary Mannich reaction to furnish the cationic intermediate B . 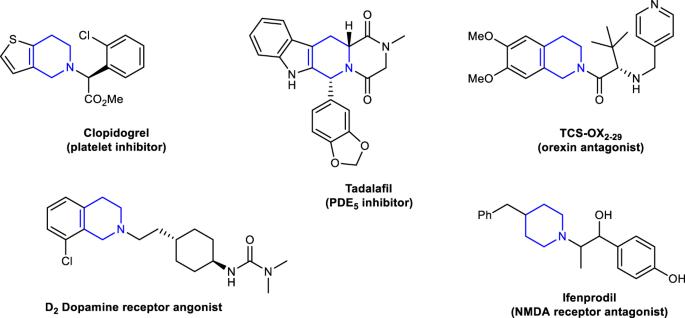Fig. 2: Pharmaceutical relevant examples of piperidines. Piperidine is widely existed in natural products and serves as the most commonly used nitrogen heterocycle among U.S. FDA-approved pharmaceuticals. Subsequently, a benzylic C−H deprotonation of B occurs to generate the dearomatized alkenyl intermediate C . C further engages in another Mannich reaction to give the cationic intermediate C2 . From C2 , the retro-Mannich reaction leads to the intermediate D , and D undergoes the intramolecular nucleophilic substitution/cyclization to furnish the benzofuran-fused piperidine derivative 4a-H . 4a-H is eventually quenched by base to provide the observed product 4a . Based on this mechanistic proposal, the electron-rich property of the benzofuran ring makes the multiple Mannich reaction and retro-Mannich reaction energetically feasible and eventually enables cyclization/alkylamination involving the benzylic C−H moiety. Consistent with this, when benzofurans with 3-(CH 2 R) substitution are used as inputs, the alkene intermediates C with poly-substituted alkene moiety are likely stabilized, thus explaining the high yields despite steric congestion ( 5n - 5r ). Fig. 6: Plausible mechanism. a Proposed mechanism. b DFT calculation. Full size image Density functional theory calculations To further explore the plausibility of our proposal, we performed a series of density functional theory (DFT) calculations. We focus on the reaction triggered by the protonation at 2-position of the benzofuran due to its prominent nucleophilicity [45] . As shown in Fig. 6b , From the intermediate int-A (which can be isolated as compd. 6 ), the Mannich reaction via TS-A is quite facile with a 5.0 kcal/mol barrier, which generates the dearomatized intermediate int-B in equilibrium. Subsequent intramolecular benzylic deprotonation proceeds via TS-B to produce the alkene intermediate int-C . This step requires a barrier of 10.7 kcal/mol ( int-B to TS-B ). From int-C , the Mannich reaction via TS-C has a 13.2 kcal/mol energy barrier and produces the intermediate int-C2 . The retro-Mannich reaction of int-C2 is quite efficient with only 1.4 kcal/mol barrier and exergonic, generating the benzofuran intermediate int-D . The final intramolecular nucleophilic substitution via TS-D allows the cyclization to give int-4a-H , which requires a barrier of 26.0 kcal/mol. Based on the additional DFT calculations, the formation of int-D is efficient and favorable. int-D is the on-cycle resting state, and the rate-determining step is the cyclization process via TS-D . These calculations validated the revised reaction mechanism, which discarded the original proposal involving the protonation of iminium intermediate. These DFT calculations revealed that the proposed reaction mechanism is rational. In summary, we have presented an unprecedented multicomponent double Mannich alkylamination for both C(sp 2 )−H and unactivated benzylic C(sp 3 )−H bonds. 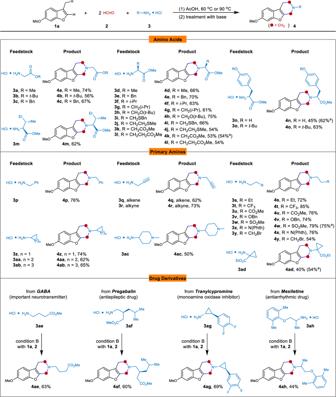Fig. 3: Substrate scope of amines. Condition A (for3a–3o):1a(0.2 mmol),2(0.8 mmol),3(0.4 mmol) in AcOH (2 mL) at 60 °C, 3 h; Condition B (for3p-3ah):1a(0.2 mmol),2(1.6 mmol),3(0.8 mmol) in AcOH (2 mL) at 90 °C, 30 mins. Yields refer to isolated products. N(Phth) =N-phthalimide.aCH3CN (2 mL) as solvent, 8 h. A series of 3-alkylbenzofurans, formaldehyde, and primary alkylamine hydrochlorides could rapidly assemble to produce the piperidines. Mechanistic studies and DFT calculations revealed a distinctive pathway that a multiple Mannich reactions and retro-Mannich reaction of benzofuran and dehydrogenation of benzylic C(sp 3 )−H bonds were key steps to constitute the alkylamination, which opens a distinctive vision for alkylamination and functionalization of unactivated C(sp 3 )−H bonds. 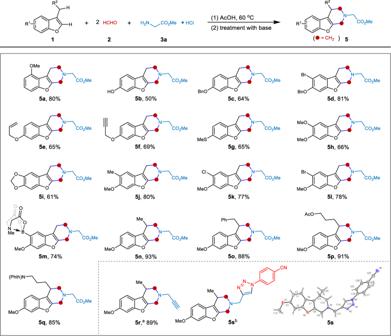Fig. 4: Substrate scope of heteroarenes. Reactions were carried out under condition A. Yields refer to isolated products. N(Phth) =N-phthalimide.a3awas replaced with propargylamine hydrochloride under condition B.b5swas prepared from5rvia click reaction. 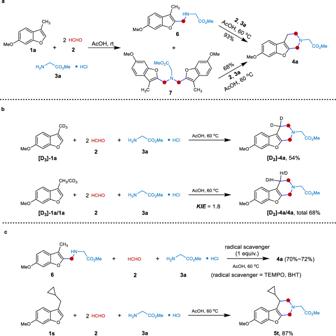Fig. 5: Mechanistic studies. aControl reaction.bKinetic isotope effect experiments.cRadical-probe experiments. 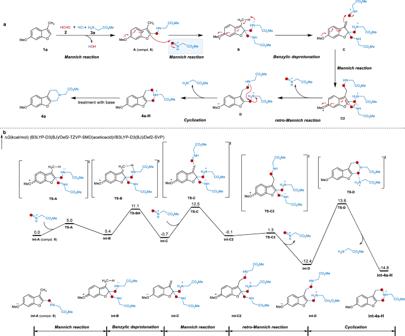Fig. 6: Plausible mechanism. aProposed mechanism.bDFT calculation. In addition, this protocol also provides a powerful tool in diversity-oriented synthesis and drug discovery.